Tolerance induction to human stem cell transplants with extension to their differentiated progeny There is increasing interest in transplantation of human stem cells for therapeutic purposes. It would benefit future application if one could achieve their long-term acceptance and functional differentiation in allogeneic hosts using minimal immunosuppression. Allogeneic stem cell transplants differ from conventional tissue transplants insofar as not all alloantigens are revealed during tolerance induction. This risks that the immune system tolerized to antigens expressed by progenitors may still remain responsive to antigens expressed later during differentiation. Here we show that brief induction with monoclonal antibody-mediated coreceptor and costimulation blockade enables long-term engraftment and tolerance towards murine ESCs, hESCs, human induced pluripotent stem cells (iPSCs) and hESC-derived progenitors in outbred murine recipients. Tolerance induced to PSC-derived progenitors extends to their differentiated progenies, and sometimes even to different tissues derived from the same donor. Global gene expression profiling identifies clear features in T cells from tolerized grafts that are distinct from those involved in rejection. The unique capacity of human pluripotent stem cells (PSCs), including the best studied embryonic stem cells (hESCs) and induced PSCs (hiPSCs), to self-renew and terminally differentiate into most cell lineages has catalysed research in tissue regeneration. Indeed, a recent report has documented the first evidence of generation of a three-dimensional, vascularized and functional human liver from hiPSCs [1] . Despite many reports describing protocols to derive a variety of cell types from hiPSCs, issues of immunogenicity remain controversial, even following ‘autologous’ transplantation [2] , [3] . Moreover, the prospect for patient-specific cell replacement therapy (CRT) seems unlikely for logistical and commercial reasons. Therefore, hESCs still remain a potentially useful cell source for CRT. Trials have been launched to study the potential therapeutic applications of hESC-derived oligodendrocyte progenitor cells [4] and hESC-derived retinal pigment epithelial cells [5] in patients with acute spinal cord injury and Stargardt’s macular dystrophy, respectively. Many more such trials are likely to be launched in the next 5–10 years [6] . We have previously demonstrated that ESC-derived tissues may exhibit an inherent degree of immune privilege that can contribute to their acceptance in allogeneic recipients [7] , [8] . This is, in part, likely due to a paucity of donor antigen-presenting cells capable of directly presenting alloantigens to T cells and absence of donor lymphocytes that can contribute to inflammation by generation of graft-versus-host reactions. In some circumstances, regulatory T cells (Treg) are also recruited or differentiated de novo from naive T cells to suppress rejection [7] , [8] , [9] , as seen in transplants of differentiated tissues in conventional organ transplantation. One would like to be able to use short-term therapies to tolerize hosts to avoid the long-term problems to both recipient and transplanted tissue associated with conventional immunosuppression. In the context of stem cell-based CRT, certain of the conventional immunosuppressants such as cyclosporine and dexamethasone can strongly inhibit terminal differentiation of neural progenitor cells into mature neurons [10] . Therefore, the ideal immunosuppressants would be those with least toxicity and least effect on cell maturation and function, yet capable of providing long-term benefit from short-term therapy; in other words, able to induce immunological tolerance. However, unlike conventional tissue grafts, ESC-derived grafts pose a novel challenge for tolerance-inducing strategies, because cells that differentiate from them will carry sets of antigens distinct from those of the parental progenitor cells. In which case, any tolerance induced to the parental progenitor cells would need to be extended to their differentiated progenies. An attractive regimen to achieve this would be the recruitment of antigen-specific Treg that could mediate bystander or linked suppression and operate throughout life by continuous harnessing further regulation through infectious tolerance [11] , [12] , [13] , [14] , a process by which tolerance is transferred from one cell population to another [14] . Although there are reports of antibody-based protocols using costimulation blockade (anti-CD40L, -LFA-1 and CTLA4Ig) that promote short-term acceptance of hESC-derived tissues in rodent model systems [15] , [16] , it is unclear whether long-term acceptance (>90 days) can be achieved, and if so, whether this could extend to tolerance of differentiated cell types derived from such stem cells. On the basis of our previous rodent studies where antibody-mediated dominant and infectious tolerance could be induced to fully allogeneic skin grafts [13] , we reasoned that combined short-term coreceptor/costimulation blockade might offer a simple route to induce acceptance of hPSC-derived tissues. Here we show that such antibody-mediated induction strategies do indeed allow long-term survival and engraftment of human xenografts in mice, in sites not acknowledged as immunologically privileged (for example, beneath the kidney capsule or within the subcutaneous space). We also demonstrate that tolerance can be induced in this way to hESC-derived progenitor cells of all three embryonic germ layers, as well as their differentiated progenies. Importantly, tolerance to hESC-derived progenitor cells, although specific to the initial inducing antigens, extended to diverse tissue types derived from the same parental stem cells presumably through regulatory mechanisms directed to common antigens expressed by both progenitor cells and their differentiated progenies that produce collateral benefit towards the differentiation-specific antigens. We sought evidence of any recruitment of T-cell reprogramming towards tolerance by analysis of global gene expression profiling on isolated T cells. The gene expression profiles of T cells infiltrating tolerized and rejecting grafts were found to be very different, likely reflecting the multiple mechanisms underlying the behaviour of tolerant and rejecting populations. Induction of graft acceptance to PSC-derived tissues We have previously reported that a combination of coreceptor (CD4 and CD8) and costimulation (CD40L) blockade was required to tolerize mice to fully histoincompatible skin grafts [13] . 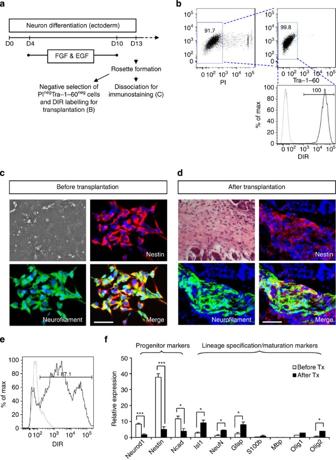Figure 1: Short-term coreceptor and costimulation blockade induces tolerance and maturation of human ESC-derived neural progenitor cells. (a) Differentiation protocol used to derive human neural progenitor cells. (b) Negative selection for PI−Tra-1-60−and positive selection for DIR+human neural progenitor cells by flow cytometry on day 13 of human ESC differentiation. (c) A representative live image and immunostaining of human neural progenitor cells with neural cell-specific markers nestin (red), neurofilament (green) and DAPI (blue) on day 13 of differentiation (n=5). Scale bar, 25 μM. (d) Frozen sections of human neural cells transplanted under the kidney capsule of CD-1 mice for 30 days following treatment with anti-CD4, -CD8 and -CD40L mAbs. Sections were stained with nestin (red), neurofilament (green) and DAPI (blue). Scale bar, 50 μM. (e) Purification of DIR+human neural cells by flow cytometry on day 30 of transplantation. (f) Quantitative RT–PCR of DIR+human neural cells on day 30 of transplantation; expression levels of the progenitor or terminally differentiated cell markers were compared with that of undifferentiated hESCs (value onyaxis=1). Data are presented as mean±s.d. *P<0.05 and ***P<0.005. While costimulation blockade alone via the anti-CD40L monoclonal antibody (mAb) was insufficient to induce transplantation tolerance [17] , coreceptor blockade alone was sufficient to induce acceptance of murine CBA/Ca ESC-derived embryoid bodies (EBs) in fully allogeneic C57Bl/6 [H-2 b ] recipients ( n =10, Table 1 ). These results expose some inherent capacity of ESC-derived tissues to benefit from therapeutic protocols for tolerance induction. To enable acceptance of xenogeneic human PSC-derived tissues, hESC-derived EBs were transplanted under the kidney capsule (not generally considered to be immunologically privileged) of outbred CD-1 mice following treatment with coreceptor and/or costimulation blockade ( Table 1 ). Unlike past experience with murine ESCs, coreceptor blockade alone was insufficient to induce tolerance to hESC-derived tissues ( n =10, Table 1 ) and no graft elements remained by the end of 30 days post transplantation. 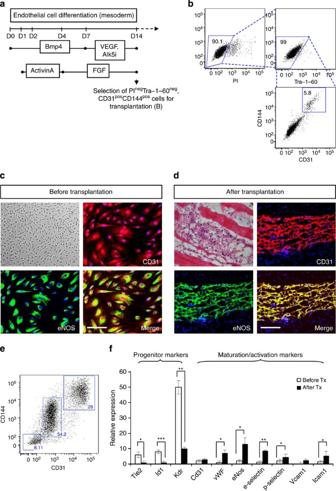Figure 2: Short-term coreceptor and costimulation blockade induces tolerance and maturation of hESC-ECs. (a) Differentiation protocol used to derive human endothelial progenitor cells. (b) Negative selection for PI−Tra-1-60−and positive selection for DIR+human endothelial progenitor cells by flow cytometry on day 13 of human ESC differentiation. (c) A representative live image and immunostaining of endothelial progenitor cells with endothelial cell-specific markers CD31 (red), eNOS (green) and DAPI (blue) on day 14 of differentiation (n=5). Scale bar, 25 μM. (d) Frozen sections of human endothelial cells transplanted under the kidney capsule of CD-1 mice for 30 days following treatment with anti-CD4, -CD8 and -CD40L mAbs. Sections were stained with CD31 (red), eNOS (green) and DAPI (blue). Scale bar, 50 μM. (e) Purification of CD31+CD144+human endothelial cells by flow cytometry on day 30 of transplantation. (f) Quantitative RT–PCR of CD31+CD144+human endothelial cells using anti-human CD31 and CD144 mAbs on day 30 of transplantation; expression levels of the progenitor or activation markers were compared with that of undifferentiated hESCs (value onyaxis=1). Data are presented as mean±s.d. *P<0.05, **P<0.01 and ***P<0.005. hESC-derived EBs were accepted ( n =30, Table 1 ) and differentiated into all three embryonic germ layers 90 days post transplantation ( n =10, Table 2 ; Supplementary Fig. 1 ) following treatment with combined coreceptor and costimulation blockade. Supplementary Figure 1b particularly demonstrates the engrafted elements following subrenal transplantation. Similarly, hiPSC-derived EBs were accepted 30 ( n =10) or 90 ( n =10) days post transplantation following treatment with both coreceptor and costimulation blockade ( Table 2 ). No graft elements could be observed in the untreated group by the end of 30 or 90 days post transplantation. Table 1 Acceptance rate of fully allogeneic or xenogeneic grafts following coreceptor and costimulation blockade. Full size table Table 2 Acceptance rate of human ESC- or iPSC-derived tissues at day 30 or 90 post transplantation following coreceptor and costimulation blockade. Full size table Induction of maturation to hESC-derived neural progenitors Since the accepted EBs formed teratomas in vivo that consisted of ectoderm-like cells ( Supplementary Fig. 1c ), we examined whether our short-term tolerizing protocol could enable acceptance of human neural progenitor cells of the ectoderm lineage. hESCs were directed to differentiate into neural progenitor cells with EGF and FGF2 using a protocol ( Fig. 1a ) modified from previous reports [18] . hESC-derived neural progenitor cells were isolated from neural rosettes and labelled with the DIR dye for human cell tracking after transplantation. These cells were also stained with propidium iodide (PI) and Tra-1-60, and the PI − DIR + Tra-1-60 − population was purified by flow cytometry to prevent contamination with PI + dead cells and formation of teratomas by Tra-1-60 + undifferentiated hESCs before transplantation ( Fig. 1b ). To confirm cell identity at the end of directed differentiation, we performed immunostaining ( Fig. 1c ) and quantitative reverse transcription PCR (RT–PCR; Fig. 1f ) to check for expression of neural progenitor cell-specific markers including nestin, neurofilament, neurogenic differentiation 1 (Neurod1) and N-cadherin (NCad). Our results confirmed that all the transplanted hESC-derived neural progenitor cells were nestin + neurofilament + before transplantation ( Fig. 1c ). The PI − DIR + Tra-1-60 − nestin + neurofilament + human neural progenitor cells were transplanted under the kidney capsule of CD-1 mice following three injections of anti-CD4, -CD8 and -CD40L mAbs within the first week post transplantation and graft acceptance was monitored at day 30, 90 and 180 post transplantation. The grafted human neural progenitor cells survived for 1 month ( n =30), 3 months ( n =10) and 6 months ( n =6) following only three doses of coreceptor and costimulation blockade in the first week post transplantation ( Table 2 ). As no graft remains could be detected in the untreated group, no further analyses could be applied at 1 month post transplantation in the control group. Figure 1: Short-term coreceptor and costimulation blockade induces tolerance and maturation of human ESC-derived neural progenitor cells. ( a ) Differentiation protocol used to derive human neural progenitor cells. ( b ) Negative selection for PI − Tra-1-60 − and positive selection for DIR + human neural progenitor cells by flow cytometry on day 13 of human ESC differentiation. ( c ) A representative live image and immunostaining of human neural progenitor cells with neural cell-specific markers nestin (red), neurofilament (green) and DAPI (blue) on day 13 of differentiation ( n =5). Scale bar, 25 μM. ( d ) Frozen sections of human neural cells transplanted under the kidney capsule of CD-1 mice for 30 days following treatment with anti-CD4, -CD8 and -CD40L mAbs. Sections were stained with nestin (red), neurofilament (green) and DAPI (blue). Scale bar, 50 μM. ( e ) Purification of DIR + human neural cells by flow cytometry on day 30 of transplantation. ( f ) Quantitative RT–PCR of DIR + human neural cells on day 30 of transplantation; expression levels of the progenitor or terminally differentiated cell markers were compared with that of undifferentiated hESCs (value on y axis=1). Data are presented as mean±s.d. * P <0.05 and *** P <0.005. Full size image To confirm cell identity at the end of study, grafts were harvested and nestin + neurofilament + human cells were observed in the graft sites 30 days post transplantation ( Fig. 1d ). It has been reported that conventional immunosuppressants such as cyclosporine and dexamethasone strongly inhibit terminal differentiation of neural progenitor cells into mature neurons [10] . To examine whether our tolerizing protocol allows terminal differentiation and maturation of the grafted human neural progenitor cells, grafts were dissociated with liberase and DIR + cells were purified by flow cytometry ( Fig. 1e ) for subsequent analyses with quantitative RT–PCR. Our human gene expression analyses showed that the grafted cells downregulated neural progenitor cell-specific genes (Neurod1, nestin, NCad) and upregulated neuron-specific genes (Isl1, NeuN), astrocyte-specific gene (Gfap) and glial cell-specific genes (Olig1, Olig2) at 30 days post transplantation compared with that of hESC-derived neural progenitor cells before transplantation ( Fig. 1f ). The gene expression pattern revealed that multiple cell lineages of the neuron system (neurons/astrocytes/glial cells) had spontaneously differentiated from the grafted human neural progenitor cells in vivo . Induction of maturation to hESC-derived endothelial progenitors Since the tolerized EBs formed teratomas in vivo that consisted of mesoderm-like cells ( Supplementary Fig. 1d ), we examined whether our tolerizing protocol could enable acceptance of human endothelial cells of the mesoderm lineage. hESCs were directed to differentiate into endothelial progenitor cells ( Fig. 2a ), modified from our previous report [19] . At the end of directed differentiation, cells were stained with PI and Tra-1-60 and with endothelial cell-specific markers, CD31 and CD144 ( Fig. 2b ). The PI − Tra-1-60 − CD31 + CD144 + hESC-derived endothelial progenitor cell (hESC-ECs) population was purified by flow cytometry to prevent contamination with PI + dead cells and formation of teratomas by Tra-1-60 + undifferentiated hESCs before transplantation ( Fig. 2b ). To confirm cell identity at the end of directed differentiation, we also performed immunostaining ( Fig. 2c ) and quantitative RT–PCR ( Fig. 2f ) to check for expression of endothelial progenitor cell-specific markers including CD31, endothelial nitric oxide synthase (eNOS), Tie2, Id1 and VEGF receptor (Kdr). Our results confirmed that all the transplanted hESC-ECs were CD31 + eNOS + before transplantation ( Fig. 2c ). The PI − Tra-1-60 − CD31 + CD144 + eNOS + hESC-ECs were transplanted subcutaneously (s.c.) into CD-1 mice following three injections of anti-CD4, -CD8 and -CD40L mAbs within the first week post transplantation and graft acceptance was monitored at day 30 and 90 post transplantation. The grafted human endothelial progenitor cells survived for at least 3 months following this brief induction protocol ( Supplementary Fig. 2 ). Figure 2: Short-term coreceptor and costimulation blockade induces tolerance and maturation of hESC-ECs. ( a ) Differentiation protocol used to derive human endothelial progenitor cells. ( b ) Negative selection for PI − Tra-1-60 − and positive selection for DIR + human endothelial progenitor cells by flow cytometry on day 13 of human ESC differentiation. ( c ) A representative live image and immunostaining of endothelial progenitor cells with endothelial cell-specific markers CD31 (red), eNOS (green) and DAPI (blue) on day 14 of differentiation ( n =5). Scale bar, 25 μM. ( d ) Frozen sections of human endothelial cells transplanted under the kidney capsule of CD-1 mice for 30 days following treatment with anti-CD4, -CD8 and -CD40L mAbs. Sections were stained with CD31 (red), eNOS (green) and DAPI (blue). Scale bar, 50 μM. ( e ) Purification of CD31 + CD144 + human endothelial cells by flow cytometry on day 30 of transplantation. ( f ) Quantitative RT–PCR of CD31 + CD144 + human endothelial cells using anti-human CD31 and CD144 mAbs on day 30 of transplantation; expression levels of the progenitor or activation markers were compared with that of undifferentiated hESCs (value on y axis=1). Data are presented as mean±s.d. * P <0.05, ** P <0.01 and *** P <0.005. Full size image To confirm cell identity at the end of study, grafts were harvested and CD31 + eNOS + human cells were observed in the graft sites 30 days post transplantation ( Fig. 2d ). To examine whether our tolerizing protocol allows terminal differentiation and maturation of the grafted human endothelial progenitor cells, grafts were dissociated with liberase and stained with anti-human (h) CD31 and hCD144 mAbs. CD31 + CD144 + cells were then purified by flow cytometry ( Fig. 2e ) for subsequent analyses with quantitative RT–PCR. Human gene expression analyses showed that the grafted cells expressed less endothelial progenitor cell-specific genes (Tie2, Id1, Kdr) but more activated and mature endothelial cell-specific genes (vwf, e-selectin, p-selectin, Vcam1, Icam1) 30 days post transplantation compared with that of hESC-ECs before transplantation ( Fig. 2f ). To examine whether our tolerizing protocol allows long-term survival of the grafted hESC-ECs, grafts were harvested and vascular structures were examined by histology 90 days post transplantation ( Supplementary Fig. 2a,b ). In addition, grafts were stained with anti-hCD31, -hCD144, -vWF and -eNOS mAbs, which are endothelial cell-specific markers ( Supplementary Fig. 2c,f ). Induction of tolerance in a tissue-specific manner We have previously shown that, within tolerant hosts, CD4 + FoxP3 + Treg are constantly vigilant in suppressing effector T cells capable of rejecting murine skin [13] . 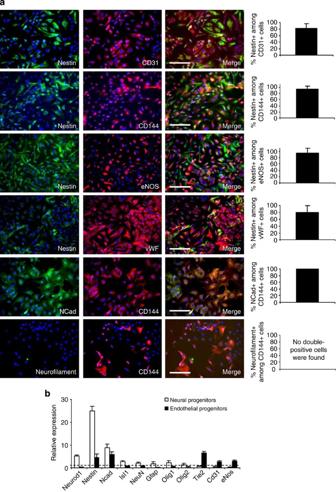Figure 3: Expression of common antigens by hESC-ECs. (a) Immunostaining of neural cell-specific markers (green) and endothelial cell-specific markers (red) expressed by CD31+CD144+endothelial progenitor cells on day 14 of human ESC differentiation (n=5). Scale bar, 50 μM. (b) Quantitative RT–PCR of neural progenitor cells or CD31+CD144+endothelial progenitor cells on days 13–14 of differentiation; expression levels of the neural cell-specific or endothelial cell-specific genes, respectively, were compared with that of undifferentiated hESCs (value onyaxis=1). Data are presented as mean±s.d. In the present study, all hESC-derived neural progenitor cells survived for at least 30 days after subcutaneous transplantion into the same CD-1 recipients that had accepted neural progenitor cells derived from the same hESC line (H9) 120 days ago ( n =6, Table 3 ). Similarly, all hESC-ECs survived for at least 30 days after subcutaneous transplantation into the same CD-1 recipients that had accepted neural progenitor cells derived from the same hESC line (H9) 120 days previously ( n =6, Table 3 ), suggesting that once tolerance had been established it was sufficient to guarantee survival of a second graft of a different tissue type derived from the same donor hESCs, without further immunosuppression. Table 3 Acceptance of human ESC-derived tissues is tissue antigen specific and maintained through ‘linked suppression’. Full size table To determine whether acceptance of hESC-ECs was a result of antigen recognition during tolerance induction to the primary neural grafts, the primary grafts were stained with both neural (nestin) and endothelial (CD31, CD144, eNOS, vWF) cell-specific antigens ( Supplementary Fig. 3 ). Importantly, the primary grafts did not express endothelial cell-specific markers that, therefore, would not have been seen during the tolerization window. To confirm that the second graft expressed a range of antigens in common with the primary graft, hESC-ECs were also stained with both endothelial (CD31, CD144, eNOS, vWF) and neural (nestin, NCad, neurofilament) cell-specific markers before transplantation ( Fig. 3a ). Intriguingly, all endothelial progenitor cells also expressed known neural progenitor cell-specific antigens nestin and NCad. It is worth noting that the same batches of antibodies were used for Figs 2 and 3 , indicating that the negative results on CD31, CD144, eNOS and vWF expression in Supplementary Fig. 3 were not due to non-functional antibodies. We performed quantitative RT–PCR to compare neural (Neurod1, nestin, Ncad, Isl1, NeuN, Gfap, Olig1, Olig2) and endothelial (Tie2, Cd31, eNos) gene expressions between neural and endothelial progenitor cells ( Fig. 3b ). Our results were consistent with that of immunostaining, which showed that endothelial cell progenitors expressed nestin and Ncad as common antigens with neural progenitor cells. This sampling of common antigens between two tissues derived from identical host hESCs allows us to propose that linked suppression towards many shared antigens, when presented on host antigen-presenting cells, could account for acceptance of the heterologous tissue types by tolerant hosts. Figure 3: Expression of common antigens by hESC-ECs. ( a ) Immunostaining of neural cell-specific markers (green) and endothelial cell-specific markers (red) expressed by CD31 + CD144 + endothelial progenitor cells on day 14 of human ESC differentiation ( n =5). Scale bar, 50 μM. ( b ) Quantitative RT–PCR of neural progenitor cells or CD31 + CD144 + endothelial progenitor cells on days 13–14 of differentiation; expression levels of the neural cell-specific or endothelial cell-specific genes, respectively, were compared with that of undifferentiated hESCs (value on y axis=1). Data are presented as mean±s.d. Full size image To examine whether the established tolerance was sufficient to maintain survival of a second graft of diverse tissue types derived from the same donor hESCs, or of the same tissue type derived from a different donor of hESCs, we have subcutaneously transplanted EBs derived from the same parental hESC line (H9) or neural progenitor cells derived from a different donor hESC line (H1) 90 days following transplantation of hESC-derived neural progenitor cells (H9). While the primary grafts remained intact 90 days following transplantation, all the H9 hESC-derived EBs and H1 hESC-derived neural progenitor cells were rejected 30 days post transplantation ( n =6 in each group, Table 3 ), suggesting that tolerance induction through coreceptor and costimulation blockade is relatively tissue antigen-specific and acceptance of the second graft depends on the types and numbers of antigen difference from the primary graft. A shift from effector T cell to Treg graft infiltration We compared the T-cell response against the tolerized xenografts derived from mAb-treated recipients versus rejecting xenografts derived from the same strain of untreated recipients. To examine whether coreceptor and costimulation blockade had an effect on the quantity and type of infiltrating T cells as an indicator of immunoregulation [7] , [8] , rejecting or tolerized neural progenitor cells were dissociated at the indicated time points with liberase and stained with CD3, CD4 or CD8 antibodies for flow cytometric analyses. Our results showed that there were more infiltrating CD3 + cells in the rejecting grafts at day 7 (4–6% of total cells, n =6) post transplantation compared with that of the tolerized grafts at day 7 (0.5–1.5%, n =6), 30 (0.5–1.3%, n =6) and 90 (2–3%, n =6) post transplantation ( Fig. 4a ). Specifically, there were also more infiltrating CD8 + cells in the rejecting grafts at day 7 (5–6%, n =6) post transplantation compared with that of the tolerized grafts at day 7 (2.5–3.5%, n =6), 30 (0.2–0.8%, n =6) and 90 (1–1.5%, n =6) post transplantation ( Fig. 4b ). Interestingly, the proportion of infiltrating CD4 + cells was greatest at an earlier time point (day 7) in both the rejecting and tolerized grafts compared with later time points (days 30 and 90) in the tolerized grafts ( Fig. 4b ), although grafts were no longer present at later time points (days 30 and 90) in the rejecting recipients. 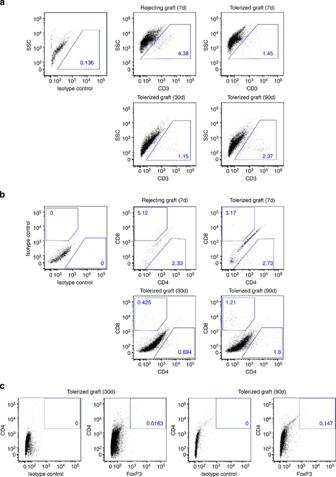Figure 4: Tolerized grafts of hESC-derived neural cells display less infiltrating effector T cells but more infiltrating regulatory T cells. (a) Representative plots of flow cytometry showing intragraft infiltration of CD3+T cells transplanted under the kidney capsule of untreated recipients (rejecting grafts) or anti-CD4, -CD8 and -CD40L mAb-treated recipients (tolerized grafts) at the indicated time point of transplantation (n=3). (b) Representative plots of flow cytometry showing intragraft infiltration of CD8+or CD4+T cells transplanted under the kidney capsule of untreated recipients or mAb-treated recipients at the indicated time point of transplantation (n=3). (c) Representative plots of flow cytometry showing infiltration of CD4+FoxP3+T cells in grafts transplanted under the kidney capsule of mAb-treated recipients at the indicated time point of transplantation (n=3). Figure 4: Tolerized grafts of hESC-derived neural cells display less infiltrating effector T cells but more infiltrating regulatory T cells. ( a ) Representative plots of flow cytometry showing intragraft infiltration of CD3 + T cells transplanted under the kidney capsule of untreated recipients (rejecting grafts) or anti-CD4, -CD8 and -CD40L mAb-treated recipients (tolerized grafts) at the indicated time point of transplantation ( n =3). ( b ) Representative plots of flow cytometry showing intragraft infiltration of CD8 + or CD4 + T cells transplanted under the kidney capsule of untreated recipients or mAb-treated recipients at the indicated time point of transplantation ( n =3). ( c ) Representative plots of flow cytometry showing infiltration of CD4 + FoxP3 + T cells in grafts transplanted under the kidney capsule of mAb-treated recipients at the indicated time point of transplantation ( n =3). Full size image To search for any possible role of tissue-infiltrating Treg in graft acceptance, the proportion of CD4 + FoxP3 + Treg in spleens (a secondary lymphoid organ) and grafts of the tolerized recipients was quantified by flow cytometry. Although FoxP3 alone might not be able to locate all Treg, we have previously demonstrated in multiple studies that FoxP3 is the most reliable marker to determine Treg localization and function [7] , [8] , [13] . As we can see in Supplementary Fig. 4 , the proportion of CD4 + FoxP3 + cells in spleens of the tolerized recipients was comparable to that of spleens of untreated mice. However, we observed infiltrating CD4 + FoxP3 + cells in the tolerized grafts at days 30 and 90 post transplantation ( Fig. 4c ). Our results were consistent with our previous studies where we found infiltrating Treg in the tolerized graft at days 30 (refs 7 , 8 ) and 90 (refs 20 , 21 ) post transplantation, suggesting that combined coreceptor/costimulation blockade may have enabled Treg to accumulate in the tolerized tissue. It is also interesting to note that there were more infiltrating CD8 + and CD4 + cells in the tolerized grafts at day 90 compared with day 30 ( Fig. 4b ), but also more CD4 + FoxP3 + Treg in the tolerized grafts at day 90 compared with that at day 30 ( Fig. 4c ) post transplantation, not inconsistent with the possibility that tissue Treg were maintaining constant vigilance in keeping the peace in the accepted tissues [13] . Gene expression profiling of tissues and CD3 + lymphocytes Certain genetic profiles have been previously described for anergic [15] , [22] and regulatory T cells [23] , [24] , [25] during the course of wound healing, autoimmunity and tolerance induction. To examine the underlying mechanisms for immune regulation during tolerance induction to hESC-derived tissues, global gene expression profiles of CD3 + cells purified from xenografts of untreated recipients (rejecting) or recipients treated with combined coreceptor and costimulation blockade (tolerized) were analysed by microarrays and quantitative RT–PCR 30 days post transplantation ( Fig. 5a ). Results from gene set enrichment analysis (GSEA) showed that the two populations were clearly different. Genes associated with a number of immunological and metabolic pathways were significantly enriched in the tolerance-associated group ( Fig. 5b ). There were 50 genes significantly upregulated ( Fig. 5c , P <0.001) and 50 others downregulated ( Fig. 5d , P <0.001), respectively, in CD3 + cells purified from xenografts of tolerized recipients compared with those of the rejecting recipients. There were genes both upregulated and downregulated by tolerized T cells in each of these pathways, suggesting a mixed population of T cells within the total CD3 + population. Specifically, CD3 + cells isolated from tolerized recipients showed a significant upregulation of genes ( P <0.05) involved in apoptosis (mitochondrial pathway), cell adhesion, mRNA destabilization (by KSRP, BRF1 or tristetraprolin) and TGFb/IL10 synthesis (intestinal immune network for IgA production) compared with that of the rejecting controls ( Supplementary Table 1a ). Also, CD3 + cells isolated from tolerized recipients showed a significant downregulation of genes ( P <0.05) involved in inflammation (4-1BB-dependent tumour-necrosis factor (TNF) receptor pathway such as NFkB, Ifng, Il2) compared with that of the rejecting controls ( Supplementary Table 1b ). 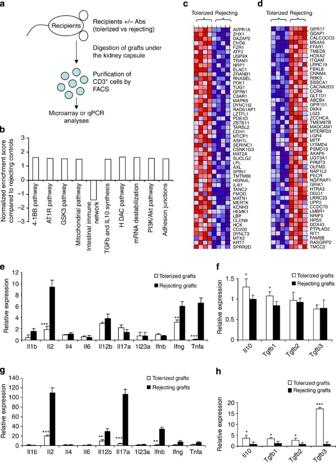Figure 5: Gene expression profiling of tissues and their infiltrating CD3+T cells during immunoregulation. (a) Schematic diagram of experimental design. (b) Results of microarray analyses showing normalized enrichment score of CD3+cells isolated from the tolerized grafts compared with that of the rejecting grafts. (c,d) Top 50 most differentially expressed genes (c) upregulated or (d) downregulated in CD3+cells isolated from the tolerized grafts compared with that of the rejecting grafts. (e,f) Quantitative RT–PCR of CD3+cells isolated from untreated recipients (rejecting grafts) or anti-CD4, -CD8 and -CD40L mAb-treated recipients (tolerized grafts) on day 30 of transplantation; their expression levels of (e) pro-inflammatory or (f) anti-inflammatory cytokines were compared with that of cells isolated from an empty matrigel plug transplanted in untreated mice to capture resting infiltrates (value onyaxis=1). (c,d) Quantitative RT–PCR of DIR+human neural cells isolated from untreated recipients (rejecting grafts) or anti-CD4, -CD8 and -CD40L mAb-treated recipients (tolerized grafts) on day 30 of transplantation; their expression levels of (g) pro-inflammatory or (h) anti-inflammatory cytokines were compared with that of undifferentiated hESCs (value onyaxis=1). Data are presented as mean±s.d. *P<0.05, **P<0.01 and ***P<0.005. Figure 5: Gene expression profiling of tissues and their infiltrating CD3 + T cells during immunoregulation. ( a ) Schematic diagram of experimental design. ( b ) Results of microarray analyses showing normalized enrichment score of CD3 + cells isolated from the tolerized grafts compared with that of the rejecting grafts. ( c , d ) Top 50 most differentially expressed genes ( c ) upregulated or ( d ) downregulated in CD3 + cells isolated from the tolerized grafts compared with that of the rejecting grafts. ( e , f ) Quantitative RT–PCR of CD3 + cells isolated from untreated recipients (rejecting grafts) or anti-CD4, -CD8 and -CD40L mAb-treated recipients (tolerized grafts) on day 30 of transplantation; their expression levels of ( e ) pro-inflammatory or ( f ) anti-inflammatory cytokines were compared with that of cells isolated from an empty matrigel plug transplanted in untreated mice to capture resting infiltrates (value on y axis=1). ( c , d ) Quantitative RT–PCR of DIR + human neural cells isolated from untreated recipients (rejecting grafts) or anti-CD4, -CD8 and -CD40L mAb-treated recipients (tolerized grafts) on day 30 of transplantation; their expression levels of ( g ) pro-inflammatory or ( h ) anti-inflammatory cytokines were compared with that of undifferentiated hESCs (value on y axis=1). Data are presented as mean±s.d. * P <0.05, ** P <0.01 and *** P <0.005. Full size image Furthermore, we performed quantitative RT–PCR to confirm gene expression profiles of pro-inflammatory and anti-inflammatory cytokines expressed by CD3 + T cells purified from xenografts of rejecting or tolerized recipients. There were significantly lower expression levels of Il2, Ifna and Tnfa ( P <0.01, Fig. 5e ), but significantly higher expression levels of Il10 and Tgfb1 ( P <0.05, Fig. 5f ) in CD3 + T cells isolated from the tolerized grafts compared with that of rejecting xenografts. Finally, to assess the overall inflammatory states of the transplanted grafts, we have also performed quantitative RT–PCR to examine gene expression profiles of pro-inflammatory, anti-inflammatory and regulatory cytokines expressed by xenografts of the rejecting or tolerized recipients. We found that there were significantly lower expression levels of genes for pro-inflammatory cytokines ( P <0.01, Fig. 5g ), particularly Il2, Il12b, Il17a and Ifna, but significantly higher expression levels of anti-inflammatory and regulatory cytokine genes ( P <0.05, Fig. 5h ), particularly Il10, Tgfb1, Tgfb2 and Tgfb3, in the tolerized xenografts compared with that of the rejecting xenografts. Although there was a slight difference in expression levels of genes between the cysts and teratomas, comparable patterns could be observed in the majority of genes of pro-inflammatory ( Supplementary Fig. 5 ), anti-inflammatory and regulatory cytokines ( Supplementary Fig. 6 ) between tolerized and rejecting xenografts of hESC-derived EBs. The critical shortage of donor organs for treating end-stage organ failure emphasizes the need for deriving tissue organs from hPSCs, predominantly hiPSCs, for transplantation. Recent advances show that a vascularized and functional human liver can be generated from hiPSCs by transplanting hiPSC-derived liver buds into immunocompromised murine recipients [1] . Although autologous transplantation with self hiPSC-derived tissues would be ideal, more work is still needed to rule out immunogenicity of such cells resulting from their reprogramming, differentiation and engraftment into autologous recipients. Nevertheless, allogeneic hESC-derived progenitor cells/tissues will likely be used for clinical transplantation, particularly in conditions involving acute injuries [4] , [5] , [19] , [26] , [27] . We have reported previously that ESC-derived tissues can acquire immune privilege by recruiting antigen-specific Treg to ensure their spontaneous acceptance across minor [8] or class-I major [7] histocompatibility barriers. This facility to acquire immune privilege likely contributes to our finding that, for the first time, a short-term antibody-based protocol has proven able to achieve long-term tolerance to hESC-derived neural or endothelial progenitor cells in murine hosts. Our protocol ensured long-term acceptance, continued differentiation and maturation of hESC-derived progenitor cells in vivo , in a xenotransplantation setting, such acceptance associated with an enhanced presence of CD4 + FoxP3 + Treg in the tolerized grafts. Although it is clearly beneficial to be able to transplant human progenitor cells capable of self-renewing or differentiating into multiple cell types of interest, hESC-derived progenitor cells pose a special challenge for tolerance induction because their diverse differentiated progenies will express different sets of lineage-specific and maturation antigens distinct from those of parental progenitor cells. For instance, we showed that the transplanted neural progenitor cells newly expressed Olig2 on 30-day differentiation in vivo ( Fig. 1f ), and transplanted endothelial progenitor cells expressed e-selectin, p-selectin, ICAM1 and VCAM1 on 30-day differentiation and activation in vivo ( Fig. 2f ). Such antigens were absent in their parental progenitor cell state before further lineage commitment [19] or activation by stimuli [28] , [29] such as cytokines or growth factors in vivo . Therefore, any tolerance induced to the parental progenitor cells would need to be extended to their differentiated progenies as a collateral benefit via linked suppression and infectious tolerance [11] , [12] , [13] , [14] , [30] . Induced or peripheral Treg (pTreg) could, in principle, mediate linked suppression and amplify themselves through infectious tolerance [31] , allowing protection of subsequent committed and more mature grafts by exploiting the same set of antigens (common antigens) expressed by both progenitor cells and differentiated progenies. In this study, we gave examples of such common antigens demonstrating that both the neural progenitor cells and their differentiated progenies expressed nestin and neurofilament and both the endothelial progenitor cells and their differentiated progenitors expressed CD31 and eNOS. Another advantage of using hPSC-derived tissues for CRT is that recipients could receive a second graft without needing additional immunosuppression, given that linked suppression would be sustained by self-renewing, antigen-specific Treg. Importantly, we demonstrated that recipients accepted a second graft of the same tissue type derived from the same donor hESCs (H9 hESC-derived neural progenitor cells) 90 days following transplantation of the primary graft (H9 hESC-derived neural progenitor cells) without additional immunosuppression, demonstrating that tolerance had been established to hESC-derived tissues by combined coreceptor and costimulation blockade. A 90-day readout was chosen to avoid residual immunosuppressive effects of the initial tolerizing treatment [13] , [14] , [32] . This is consistent with our previous findings that tolerance to murine skin grafts required continous availabilty of donor antigens to maintain it [14] , [33] . In the present study, we performed a series of transplants with different sources of secondary grafts to further determine the extent to which tolerance induced to the primary graft could also protect a secondary graft of a different tissue type derived from the same donor hESCs, a combination of different tissue types derived from the same donor hESCs, or the same tissue type derived from an unrelated donor. Our data indicate that tolerance can be extended to a secondary graft of a different tissue type derived from the same donor hESCs, but not from a different major histocompatibility complex (MHC)-mismatched donor. When recipients were tolerized to H9 hESC-derived neural progenitor cells (primary graft), H9 hESC-derived endothelial cells (second graft) could also survive for at least 30 days without any additional immunosuppression. We have demonstrated that the primary neural graft does not express certain antigens considered unique to the subsequent endothelial graft. Therefore, antigens of the second graft should not have been recognized during tolerance induction to the primary graft; however, the second endothelial graft did express some antigens in common with the primary neural graft, for example, nestin and NCad. Antigens such as these might provide the basis for linked suppression extending to the unique antigens. It is conceivable that our data could be explained by the primary graft having retained a minor pluripotent population, which could theoretically have provided a source of diverse cell types and their tissue-specific antigens, during the phase of tolerance induction. In such a scenario, the second graft would have been accepted as its antigens should have been recognized during the tolerization phase. Against this though, tolerized hosts rejected secondary grafts of a combination of tissue types derived from the same donor hESCs (H9 hESC-derived EBs), indicating that they could not be tolerant to all H9 hESC-derived antigens. The host also rejected a secondary graft of the same tissue type derived from a histoincompatible allogeneic donor (H1 hESC-derived neural progenitor cells), indicating that they still had the ability to reject xenogeneic antigens and that there was an element of antigen specificity to tolerance. If, as we think, tolerance is mediated through linked suppression, then any collateral benefit would be dependent on the degree of similarity in the type and amount of antigens expressed by both the primary and secondary grafts. To determine the underlying mechanisms of tolerance induction to hESC-derived tissues by coreceptor and costimulation blockade, CD3 + T cells were isolated from tolerized (treated) or rejecting (untreated) grafts for global gene expression analyses. Our results might indicate that a mixed population of CD3 + T cells was present in the tolerant group, one expressing anti-apoptotic (upregulation of Bcl2 and downregulation of Bak or Bid) and the other expressing pro-apoptotic genes (upregulation of caspases). In general, we found that certain pathways appeared to be associated with tolerance compared with that of the rejecting controls: CD3 + cells isolated from tolerized recipients showed a significant upregulation of genes involved in apoptosis, cell adhesion and mRNA destabilization via epigenetic regulation, and syntheses of anti-inflammatory cytokines such as TGFb and IL10 ( P <0.05). On the other hand, CD3 + cells isolated from tolerized recipients showed a significant downregulation of genes involved in inflammation, particularly the 4-1BB-dependent TNF receptor pathway (NfKB, Tnfa Ifng, Il2; P <0.05). In addition to CD3 + cells within the grafts, we have also performed tissue cytokine profiling with the tolerized or rejecting grafts and found that tolerized tissues expressed lower levels of pro-inflammatory (Il2, Il12b, Il17a, Ifng) but higher levels of anti-inflammatory and regulatory cytokines (Tgfb1, Tgfb2, Tgfb3 and Il10) compared with that of the rejecting grafts ( P <0.05). Interestingly, the tolerized tissues predominantely expressed Tgfb3, while CD3 + cells predominantely expressed Tgfb1 and Il10 as protective cytokines consequent to tolerance induction. Our results were also consistent with our previous findings that hESC-derived tissues expressed Tgfb3, perhaps reflecting an additional privilege-associated mechanism contributing to the induction de novo of pTreg [7] , [8] . Foxp3 + Treg are essential for self-tolerance as multiple autoimmune diseases develop in their absence [34] . In certain circumstances where tolerance is induced therapeutically, Treg have been shown to be constantly required to suppress effector T cells that are otherwise capable of causing tissue damage [13] . Foxp3 + Treg have been shown to be empowered to maintain tolerance achieved by coreceptor and/or costimulation blockade across all levels of histocompatibility mismatch: full MHC [13] , a single MHC [7] , multiple minor [35] and a single minor [8] , [21] antigen in allogeneic murine recipients. In one study, we have also shown that coreceptor blockade induced tolerance to rat xenografts in murine recipients [36] . Nevertheless, to our knowledge, this is the first demonstration of tolerance induction to xenogeneic hESC-derived tissues by coreceptor and costimulation blockade. This might be expected if we assume the bulk of antigen presentation for regulation was indirect [9] , [30] , giving new insights into tolerance induction to xenogeneic stem cell transplantation. Strategies capable of harnessing Treg in man could then be of value to promote acceptance of human stem cell transplants. Although the equivalent coreceptor and costimulatory antibodies are not yet licensed for clinical use, there are other similar approaches to selectively harness Treg that may be of more immediate clinical relevance. For example, the more established mixed chimerism approach pioneered by Sachs and Sykes [37] has already provided some evidence that Treg may be contributing to graft acceptance, at least in some patients. Similarly, lymphocyte depletion with agents such as alemtuzumab, followed by short-term antibody therapy to guide reconstitution of the repopulating cells could also offer a clinically applicable approach [38] . Moreover, recent advances in developing drug-minimization protocols by the use of alemtuzumab combined with a short period of costimulation blockade via belatacept and mTOR inhibition promote acceptance of renal grafts without impediment to Treg function in man [39] . Nevertheless, the current study focused on the competing role(s) of effector T cells and Treg during tolerance induction to stem cell grafts. Our results highlight the need for further mechanistic studies to fully explain mechanisms of linked suppression and acquired privilege that operate in this form of therapeutic tolerance. In summary, our pre-clinical findings suggest that development of tolerizing protocols for regenerative medicine and CRT should focus on patient-friendly ways of exploiting Treg, in a manner that ensures continued differentiation and maturation of human stem cell grafts following establishment of transplantation tolerance. Mouse ESC cultures and EB differentiation The ESF116 ESC line was derived from male CBA/Ca mice as reported previously [7] . ESF116 ESCs were maintained in ES medium containing Dulbecco’s Modified Eagle’s Medium (Cambrex Bio Science Verviers), 15% v/v fetal calf serum (FCS; Gibco), 50 μg ml −1 penicillin and streptomycin, 1 mM sodium pyruvate, 2 mM L -glutamine and 50 μM 2-mercaptoethanol. Before differentiation, ESCs were passaged twice on gelatin and cultured in ES medium supplemented with 1,000 U ml −1 recombinant leukaemia inhibitory factor (rLIF; Millipore). EBs were formed from 500 ESCs per 20 μl in hanging drop cultures in the absence of rLIF for 2 days and individual EBs were then transferred to suspension cultures for another 12 days before transplantation. Human ESC cultures and lineage-specific differentiation The H9 human ESC (Wicell) and human iPSC lines (a gift from Dr Gustavo Mostoslavsky, Department of Medicine, Boston University, USA) were maintained in mTseR1 medium (Stemgent). hESCs were differentiated into derivatives of the three embryonic germ layers by stepwise administration of growth factors as described previously [18] , [19] . Briefly, for neural cell induction, hESCs were grown in clusters with neural differentiation medium containing 50% Neurobasal, 50% DMEM/F12, 2% B27 and 1% N2 (Gibco) for 4 days. Small clumps of neuroectodermal spheres were then cultured with 20 ng ml −1 FGF2 and 20 ng ml −1 EGF (R&D) for 6 days. After that, the spheres were replated on 10 μg ml −1 laminin-coated plates and cultured for 3 days to form rosettes. For endothelial cell induction, hESCs were cultured with hESC differentiation medium containing DMEM/F12, 10% knockout serum replacement (KOSR), 1 × non-essential amino acids, 1 × glutamine, 1 × penicillin/streptomycin and 1 × b-mercaptoethanol (Gibco) for 4 days. The differentiated cells were then replated in matrigel-coated plates and cultured in hESC differentiation medium containing 1% KOSR for 10 days under hypoxia (5% oxygen). A combination of growth factors was supplemented as follows: 20 ng ml −1 BMP4 (R&D, day 0–7), 10 ng ml −1 activinA (R&D, day 1–4), 10 ng ml −1 FGF2 (Peprotech, day 4–14) and 100 ng ml −1 VEGF-A (Peprotech, day 7–14). For EB induction, hESCs or hiPSCs were resuspended in hESC differentiation medium containing 10% KOSR in hanging drop cultures for 2 days. Individual EBs were then transferred to suspension cultures and incubated in hESC differentiation medium containing 1% KOSR for another 12 days before transplantation. Preparation of cells for transplantation To generate cells for transplantation, single cells were isolated using 0.25% trypsin-EDTA and stained with PI (BD) to exclude dead cells. hESC-derived neural cells were stained with fluorochrome-conjugated anti-Tra-1-60 antibody (BD, dilution 1:100) and purified on FACS AriaII (BD) to exclude the undifferentiated pluripotent stem cells. The purified PI − Tra-1-60 − cells were then labelled with DIR dye (Invitrogen) for human cell tracking according to the manufacturer’s instructions. hESC-ECs were stained with fluorochrome-conjugated anti-hCD31 and anti-hCD144 antibodies (BD, dilution 1:100) and the PI − CD31 + CD144 + cells were purified on FACS AriaII (BD). A list of antibodies used in flow cytometry is shown in Supplementary Table 2 . Kidney capsule transplantation All animal procedures were performed in accordance with protocols approved by University of Oxford or Harvard Medical School. EBs (3–5) or 5 million hESC-derived neural cells were transplanted under the kidney capsule of 12-week-old, female CD-1 mice (Charles River Laboratories International) as described previously [7] . For studying the human gene expression profiles ( Fig. 2f ), the PI − DIR + cells were purified by flow cytometry for subsequent qRT–PCR or microarray analyses. In vivo matrigel plug assay and matrigel cytometry Flow cytometry-purified, 5 million PI − CD31 + CD144 + hESC-ECs were resuspended in matrigel and injected s.c. into the 12-week-old, female CD-1 mice. Matrigel plugs were harvested at the indicated time points and hESC-ECs were isolated by flow cytometry as described previously [40] . Briefly, matrigel plugs were incubated in PBS supplemented with 25 μg ml −1 DNase (Sigma), 3 U ml −1 dispase and 3 ng ml −1 liberase (Roche) for an hour at 37 °C. The isolated cells were filtered through a 40-μm nylon mesh (BD) and washed three times with PBS. Isolated cells were then stained with fluorochrome-conjugated anti-hCD31 and anti-hCD144 antibodies and PI − CD31 + CD144 + hESC-ECs were purified from the grafts on FACS AriaII (BD). For studying the human gene expression profiles ( Fig. 2f ), the PI − CD31 + CD144 + cells were also purified by flow cytometry for subsequent qRT–PCR or microarray analyses. Administration of therapeutic antibodies Generation of anti-CD4, -CD8 and -CD40L mAbs was described previously [35] , [41] , [42] . Non-depleting mAb specific for CD4 (1 mg, clone YTS 177.9) and CD8 (1 mg, clone YTS 105.18) were injected intraperitoneally (i.p.) on days 0, 2 and 4 post transplantation of murine ESC-derived EBs. Similarly, non-depleting mAb specific for CD4 (1 mg, clone YTS 177.9), CD8 (1 mg, clone YTS 105.18) and CD40L (1 mg, clone MR1) were injected i.p. on days 0, 2, 4 and 6 after transplantation of hESCs, hiPSCs, hESC-derived neural cells or ECs. In the antigen specificity study, tolerized mice were transplanted with a second graft ( Table 3 ) 3 months after the primary grafts had been transplanted. The 3 months allowed for complete clearance of the therapeutic antibodies as previously described [32] , [35] . Immunostaining Tolerized mice were anaesthetized and perfused intracardially with 4% paraformaldehyde/PBS. Perfused kidney grafts or matrigel plugs were dissected and further fixed in 4% paraformaldehyde at 4 °C for 4 h. The fixed grafts were washed three times with PBS and equilibrated in 30% sucrose before freezing and cryosectioning. Six micrometre sections were blocked in 2% goat serum and then stained with different primary antibodies in 10 μg ml −1 at 4 °C overnight. A list of primary antibodies used is shown in Supplementary Table 1 . Alexa-Fluor-488- or Alexa-Fluor-594-conjugated secondary antibodies (Molecular Probes) were also used for unconjugated primary antibodies at room temperature for 30 min in the dark. Slides were mounted with DAPI (4',6-diamidino-2-phenylindole)-containing fluorescence mounting medium (Dako) and fluorescence was detected with a fluorescence microscope (Zeiss). Sections of each lineage were also stained with hematoxylin and eosin for histological analyses. A list of antibodies used in immunostaining is shown in Supplementary Table 2 . RNA isolation and gene expression analyses Total RNA was isolated from purified cells of both the untreated and mAb-treated groups using the RNeasy mini kit (Qiagen) and reverse transcribed using Superscript III RT (Invitrogen), according to the manufacturer’s instructions. Real-time quantitative PCR profiling was analysed on Mastercycler realplex 4 Sequence Detector (Eppendoff) via SYBR Green (QuantitectTM SYBR Green PCR Kit, Qiagen). The relative gene expression level of each sample was expressed as a relative quantitation value determined by the 2 −dd C T method, which represents the fold change in gene expression normalized to that of a housekeeping gene, Gapdh. The relative gene expression level of each sample was also compared with internal controls as indicated where appropriate. A list of complementary PCR primer sequences used is shown in Supplementary Table 3 . Microarrays and functional annotation Total RNA was isolated from purified CD3 + cells of both the untreated and mAb-treated groups using the RNeasy mini kit (Qiagen). RNA was then hybridized to the Affymetrix Mouse 430_2 chips and expression data were analysed with the GeneSpring GX 10.0 software according to the manufacturer’s instructions. The normalized data (that is, relative to housekeeping genes) were further analysed for functional annotation using GSEA as described previously [43] , [44] . GSEA examines whether a defined set of genes or ‘gene sets’ are significantly enriched at the top or bottom of a ranked list of genes from microarray experiments, which represent two phenotypes: rejecting control samples and antibody-treated samples. Gene sets including KEGG, Reactome and Biocarta symbols and the GSEA default settings were employed in this study. The microarray data have been deposited in the NCBI Gene Expression Omnibus with an accession number GSE61867. Statistical analyses The data were expressed as arithmetic mean±s.d. of biological triplicate determinations performed under the same conditions. Statistical analysis was performed using the Student’s t -test (* P <0.05, ** P <0.01 and *** P <0.001). How to cite this article: Lui, K. O. et al . Tolerance induction to human stem cell transplants with extension to their differentiated progeny. Nat. Commun. 5:5629 doi: 10.1038/ncomms6629 (2014).